An ultra-low-input native ChIP-seq protocol for genome-wide profiling of rare cell populations Combined chromatin immunoprecipitation and next-generation sequencing (ChIP-seq) has enabled genome-wide epigenetic profiling of numerous cell lines and tissue types. A major limitation of ChIP-seq, however, is the large number of cells required to generate high-quality data sets, precluding the study of rare cell populations. Here, we present an ultra-low-input micrococcal nuclease-based native ChIP (ULI-NChIP) and sequencing method to generate genome-wide histone mark profiles with high resolution from as few as 10 3 cells. We demonstrate that ULI-NChIP-seq generates high-quality maps of covalent histone marks from 10 3 to 10 6 embryonic stem cells. Subsequently, we show that ULI-NChIP-seq H3K27me3 profiles generated from E13.5 primordial germ cells isolated from single male and female embryos show high similarity to recent data sets generated using 50–180 × more material. Finally, we identify sexually dimorphic H3K27me3 enrichment at specific genic promoters, thereby illustrating the utility of this method for generating high-quality and -complexity libraries from rare cell populations. Chromatin immunoprecipitation followed by next-generation sequencing (ChIP-seq) is a widely used approach to study genome-wide DNA–protein interactions. While such experiments have yielded significant insights, standard ChIP-seq protocols require ~10 7 cells [1] , [2] , [3] , precluding their use on rare cell populations. In recent years, scaled-down ChIP-Chip [4] and ChIP-seq procedures [5] , [6] , [7] , [8] , [9] , [10] were developed for inputs ranging from 10 3 to 10 6 cells. However, most include crosslinking (XChIP) and pre-amplification of ChIP material before library construction [5] , [6] , [7] , which can reduce library complexity and generate PCR artefacts [11] . Despite advances, few groups have generated high-quality data from rare in vivo cell populations using these methods. Three groups recently published data sets from purified primordial germ cells (PGCs) pooled from the gonadal ridges of mouse embryos [10] , [12] , [13] . The large amount of input material used in these analyses, however, is prohibitive for studies involving single embryos or very rare cell types. The reduced number of steps and improved resolution relative to XChIP makes micrococcal nuclease (MNase)-based ‘native’ ChIP (NChIP) an attractive alternative to study histone modifications in rare cells. A low-input NChIP-seq method to generate high-quality and resolution-sequencing libraries was recently described [8] , but libraries built from <10 5 cells using this method had low levels of complexity and high levels of duplicates. We therefore sought to develop an improved NChIP procedure that would generate high-complexity libraries from significantly smaller amounts of input material. Here, we present a flexible and robust ultra-low-input (ULI) NChIP-seq method optimized for chromatin isolated from as few as 10 3 cells. H3K9me3 and H3K27me3 NChIP-seq libraries generated from 10 3 to 10 5 mouse embryonic stem cells (ESCs) yield results comparable to those previously generated from 10 6 ESCs. We further validated our approach by generating sex-specific H3K27me3 NChIP-seq data sets from 10 3 PGCs isolated from the gonadal ridges of single male and female E13.5 embryos. The maps generated have higher complexity and resolution than previously published data sets [12] , [13] . Moreover, by intersecting our NChIP-seq data sets with RNA-seq libraries generated from 10 3 male and female E13.5 PGCs, we identified a subset of genes involved in meiosis and transforming growth factor-β receptor signalling that show sex-specific differences in expression and H3K27me3 enrichment in their promoter regions. Complexity of ULI-NChIP-seq libraries from 10 3 to 10 5 cells To improve the yield of chromatin isolated from small samples, we optimized a dilution-based NChIP-seq procedure that can easily be adjusted to cell sample size. A comparison of our method with standard NChIP-seq and low-input XChIP-seq protocols highlighting steps improved to prevent sample loss is presented in Fig. 1a . ULI-NChIP-seq allows for sorting of cells directly into a detergent-based nuclear isolation buffer, thereby enabling extended sample storage or pooling of samples. Importantly, unlike most low-input XChIP-seq methods, no pre-amplification of ChIP material is required before library construction, minimizing the generation of PCR artefacts. 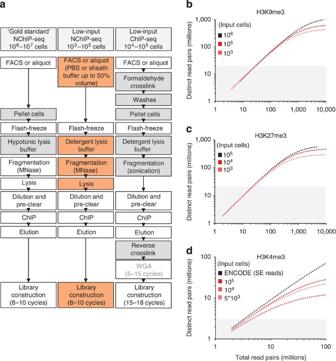Figure 1:A NChIP-seq protocol togenerate genome-wide chromatin maps from low cell numbers. (a) Overview of our improved ULI-NChIP-seq protocol and comparison with previously published NChIP-seq and low-input ChIP-seq protocols. Grey: steps associated with sample loss; orange: steps optimized to minimize sample loss. Extrapolation15of H3K9me3 (b), H3K27me3 (c) and H3K4me3 (d) library complexity based on low-input and standard ChIP-seq libraries sequenced with various depth. SE reads, single-end reads. Figure 1: A NChIP-seq protocol to generate genome-wide chromatin maps from low cell numbers. ( a ) Overview of our improved ULI-NChIP-seq protocol and comparison with previously published NChIP-seq and low-input ChIP-seq protocols. Grey: steps associated with sample loss; orange: steps optimized to minimize sample loss. Extrapolation [15] of H3K9me3 ( b ), H3K27me3 ( c ) and H3K4me3 ( d ) library complexity based on low-input and standard ChIP-seq libraries sequenced with various depth. SE reads, single-end reads. Full size image Using this protocol, we prepared H3K9me3 NChIP-seq libraries from 10 3 –10 5 ESCs ( Supplementary Fig. 1a and Supplementary Methods ). To serve as a reference, we also generated an H3K9me3 library from 10 6 ESCs using a previously described NChIP-seq (‘gold-standard’) protocol [14] . All libraries were indexed, pooled and paired-end sequenced (100 bp reads). Depending on the number of libraries pooled on a single lane, we obtained from 45–145 million reads. We evaluated library complexity by comparing the total number of distinct reads with the number of duplicate and unaligned reads in each library ( Supplementary Fig. 1b ). Unmapped reads represented from 7 to 15% of all reads, independent of sequencing depth or input size, suggesting that the low number of PCR cycles (8–10) used for library amplification introduced relatively few PCR artefacts. The H3K9me3 library prepared from 10 6 cells was sequenced the deepest (~147 million reads) and also had the highest proportion of duplicates (28%). Independent of sequencing depth (45–100 million reads) or the number of input cells, ULI libraries prepared from 10 3 to 10 5 cells had a total of 21–25% uniquely and multi-aligned duplicate reads, suggesting that these libraries were sufficiently complex for deeper sequencing ( Supplementary Fig. 1a ). As we are comparing libraries with different sequencing depths, we used the PreSeq package [15] to extrapolate and compare the potential complexity of our libraries ( Fig. 1b ). Although our H3K9me3 libraries built from 10 3 to 10 5 cells display a lower potential complexity than our ‘gold-standard’ library ( Fig. 1b , top panel), all could potentially be sequenced several times deeper than the ~20 million distinct reads recommended to generate high-quality profiles for such broad chromatin marks. In addition, we prepared H3K27me3 NChIP-seq libraries from 10 3 to 10 5 ESCs using similar conditions, and obtained 29–42 million distinct reads per library, with ~10% unmapped reads and only 3–8% total duplicate reads in each case ( Supplementary Fig. 1c ). As for H3K9me3 libraries, using PreSeq [15] to extrapolate the potential complexity of these libraries indicates that even with the lowest input, all of the H3K27me3 libraries could be several times the required depth to obtain high-quality profiles ( Fig. 1c ). To determine whether this method can be used to create profiles for active histone marks, we next generated ULI-NChIP-seq data for H3K4me3. As this promoter-enriched chromatin mark is less abundant than H3K9me3 and H3K27me3, H3K4me3 libraries were amplified for 2–4 additional PCR cycles in order to obtain sufficient material for sequencing ( Supplementary Fig. 1a ). Deep sequencing (37.7 million reads) of an H3K4me3 library built from 10 5 cells showed under 10% of unaligned reads and 36% total duplicate reads ( Supplementary Fig. 1d ). Shallow sequencing of H3K4me3 libraries prepared from 5 × 10 3 and 1 × 10 4 cells (9.5 and 7.8 million reads, respectively) showed an increased proportion of unaligned reads (55–70%), indicative of lower complexity libraries. As this was a shallow round of sequencing, the proportion of duplicate reads remains very low (<5%). Extrapolation of potential library complexity indicates that, despite the increased proportion of unaligned reads, deeper sequencing of these libraries could generate enough reads to saturate H3K4me3 peaks ( Fig. 1d ). Correlation between ULI and standard ChIP-seq libraries Visual inspection of NChIP-seq profiles from randomly chosen regions shows similar enrichment in libraries built from 10 3 to 10 6 cells ( Fig. 2a–c ). We compared H3K9me3 enrichment in genome-wide 2 kb bins, and calculated Pearson correlation coefficients to assess the similarity between ULI and standard NChIP-seq libraries ( Fig. 2d and Supplementary Fig. 2a ). H3K9me3 libraries built from 10 3 to 10 5 cells had correlations ranging from 0.83 to 0.9 when compared with ‘gold-standard’ H3K9me3 NChIP-seq. As expected, low-input libraries had modestly higher background levels, as illustrated by an increase in variance ( Supplementary Fig. 2c ). We next defined regions enriched for H3K9me3 using MACS (see Methods section). Of all H3K9me3 peaks identified in our ‘gold-standard’ library, 76–85% were also detected in libraries generated from 10 3 to 10 5 cells ( Supplementary Fig. 3a,c ). Consistent with previous reports showing that specific endogenous retroviruses (ERVs) are marked and silenced by H3K9me3 (refs 1 , 16 , 17 ), our ‘gold-standard’ and ULI libraries show H3K9me3 enrichment at the same subset of ERV1 and ERVK subfamilies ( Supplementary Fig. 4a ), in the unique 1 kb 5′ flank of ERVKs ( Supplementary Fig. 4b ), and at individual IAP ERVK elements ( Supplementary Fig. 4c ). 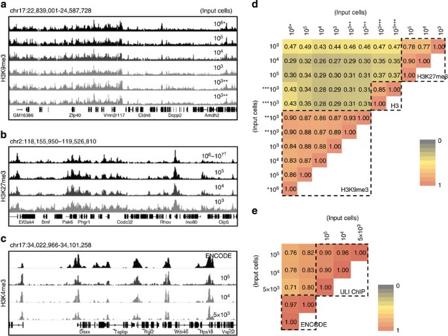Figure 2:Correlation between standard and ULI-NChIP-seq libraries built from 103to 105ESCs. Genome browser screenshots of H3K9me3 (a), H3K27me3 (b) or H3K4me3 (c) profiles at the indicated genomic locations. (d) Genome-wide Pearson correlation (50,000 random 2 kb bins) between H3K9me3, H3 and H3K27me3 enrichment (RPKM) in data sets generated from 103to 106cells as input material. *Library prepared using the ‘gold-standard’ NChIP-seq protocol. ** and ***Technical replicates.†Obtained from ref.35. (e) Pearson correlation of H3K4me3 enrichment (RPKM) around genic promoters (RefSeq TSS ±500 bp) between ULI-NChIP-seq libraries generated from 5 × 103to 5 × 105cells and ENCODE libraries18in E14 mouse ESCs. Figure 2: Correlation between standard and ULI-NChIP-seq libraries built from 10 3 to 10 5 ESCs. Genome browser screenshots of H3K9me3 ( a ), H3K27me3 ( b ) or H3K4me3 ( c ) profiles at the indicated genomic locations. ( d ) Genome-wide Pearson correlation (50,000 random 2 kb bins) between H3K9me3, H3 and H3K27me3 enrichment (RPKM) in data sets generated from 10 3 to 10 6 cells as input material. *Library prepared using the ‘gold-standard’ NChIP-seq protocol. ** and ***Technical replicates. † Obtained from ref. 35 . ( e ) Pearson correlation of H3K4me3 enrichment (RPKM) around genic promoters (RefSeq TSS ±500 bp) between ULI-NChIP-seq libraries generated from 5 × 10 3 to 5 × 10 5 cells and ENCODE libraries [18] in E14 mouse ESCs. Full size image Similarly, H3K27me3 libraries built from 10 4 to 10 5 cells were highly correlated, with a genome-wide correlation (2 kb bins) of 0.9. Likely owing to a modest increase in background levels, the library built from 10 3 cells had correlations of 0.77 and 0.78 to the libraries built from 10 4 and 10 5 cells, respectively ( Fig. 2d and Supplementary Fig. 2b,c ). Regardless, H3K27me3-enriched regions showed good correlation between libraries, with 80% and 70% of peaks detected in our 10 5 cell input library overlapping with peaks detected in our libraries built from 10 4 and 10 3 cells, respectively ( Supplementary Fig. 3b,d ). We next compared H3K27me3 enrichment levels around transcription start sites (TSSs), as H3K27me3 marks the promoter regions of bivalent or silenced genes [1] . Libraries from all input sizes showed high correlation to each other (0.86–0.96), and H3K27me3 enrichment at gene promoters was correlated with relatively low levels of gene expression, as expected ( Supplementary Fig. 5a–c ). As H3K4me3 is a narrow chromatin mark present at the promoter region of actively transcribed and bivalent genes, we compared H3K4me3 enrichment around TSSs (±500 bp) of ULI-NChIP-seq to ENCODE [18] libraries (built from E14 ESCs). We obtained high Pearson correlation coefficients between our libraries built from 5 × 10 3 to 5 × 10 5 cells (0.90–0.96) and good correlations (0.71–0.83) to ENCODE libraries ( Fig. 2e ). The lower correlations to ENCODE libraries are presumably due in part to the large difference in sequencing depth, as well as to the different ESC lines and antibodies used. Visual inspection of ChIP-seq profiles reveals that the same promoters are generally marked, but with varying intensities ( Fig. 2c ). While preliminary attempts to generate H3K4me3 profiles from 10 3 cells did not yield sufficient coverage (data not shown), further optimization of the ChIP conditions for this mark will likely improve the resolution of signal above background. Sex-specific H3K27me3 profiles in PGCs from single embryos As low-input methods are particularly useful for the study of cell types present in limited numbers in vivo , we validated our method on PGCs, the precursors to mature gametes. To determine sex-specific H3K27me3 profiles correlation to sex-specific gene expression, we used ULI-NChIP-seq data sets prepared from 10 3 PGCs purified from the gonads of single male and female E13.5 embryos [19] . Comparison with previously published low-input H3K27me3 data sets generated from 5.2 × 10 4 to 1.8 × 10 5 PGCs in two independent studies [12] , [13] reveals that our method yielded similar or greater sequencing depth while minimizing total duplicate generation (<15%) ( Fig. 3a ). Of note, while a fraction of the reads labelled as duplicates are likely owing to preferred MNase cleavage sites, the use of paired-end rather than single-end sequencing for ULI-NChIP-seq allows for improved discrimination between technical (PCR) and biological duplicate reads. While H3K27me3 enrichment patterns around and upstream of the HoxC cluster are broadly similar to those described by Ng et al . [13] and Lesch et al . [12] ( Fig. 3b ), our method yields higher resolution maps, likely owing to a combination of high number of distinct reads, longer reads and lower number of PCR amplification cycles used during library construction. In addition, fragmentation of chromatin using MNase generates smaller and more uniformly sized fragments than does sonication of crosslinked chromatin, while the use of paired-end sequencing allows for the determination of true fragment size. Relative H3K27me3 enrichment around all annotated TSSs (±2 kb) was similar to previously published data [12] , [13] ( Fig. 3c ), with Pearson correlations between 0.68 and 0.85. Of note, the more deeply sequenced of the two female libraries from Lesch et al . [12] showed greater correlation to the female H3K27me3 data set generated using ULI-NChIP-seq19 (0.69) than to its replicate library (0.51) ( Fig. 3c ). 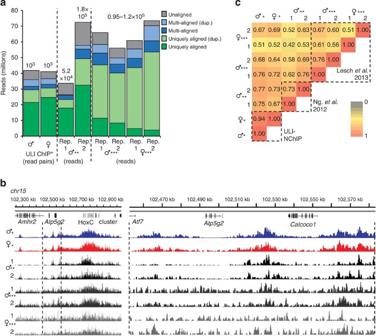Figure 3: High-resolution gender-specific H3K27me3 profiles generated from E13.5 PGCs isolated from single embryos. (a) Library complexity of H3K27me3 data sets prepared from E13.5 PGCs using ULI-NChIP-seq compared with previously published data sets generated using alternative low-input XChIP-seq protocols (*ref.13; **ref.13; ***ref.12). The number of input cells is indicated above each bar. (Rep.: Repeat) (b) Genome browser screenshots of H3K27me3 enrichment around the HoxC cluster illustrating the complexity of libraries generated using ULI-NChIP-seq library and correlation to previously published data sets12,13generated using an alternative low-input ChIP-seq protocol (*ref.13; **ref.13; ***ref.12). (c) Pearson correlations between H3K27me3 data generated from 103male PGCs using our low-input protocol and previously published data around gene promoters (RefSeq TSS ±2 kb). (*ref.13; **ref.13; ***ref.12). Figure 3: High-resolution gender-specific H3K27me3 profiles generated from E13.5 PGCs isolated from single embryos. ( a ) Library complexity of H3K27me3 data sets prepared from E13.5 PGCs using ULI-NChIP-seq compared with previously published data sets generated using alternative low-input XChIP-seq protocols (*ref. 13 ; **ref. 13 ; ***ref. [12] ). The number of input cells is indicated above each bar. (Rep.: Repeat) ( b ) Genome browser screenshots of H3K27me3 enrichment around the HoxC cluster illustrating the complexity of libraries generated using ULI-NChIP-seq library and correlation to previously published data sets [12] , [13] generated using an alternative low-input ChIP-seq protocol (*ref. 13 ; **ref. 13 ; ***ref. [12] ). ( c ) Pearson correlations between H3K27me3 data generated from 10 3 male PGCs using our low-input protocol and previously published data around gene promoters (RefSeq TSS ±2 kb). (*ref. 13 ; **ref. 13 ; ***ref. [12] ). Full size image Intriguingly, while male and female E13.5 PGCs have distinct differentiation programs and transcription patterns [12] , [20] , [21] , our results indicate that their H3K27me3 distribution profiles are broadly similar ( Supplementary Fig. 6 and ref. 19 ). Using our ULI-NChIP-seq data sets, we therefore sought to identify sex-specific H3K27me3-marked promoters associated with gene silencing in E13.5 PGCs. In both males and females, H3K27me3 around TSSs was associated with low levels of transcription ( Fig. 4a,b and ref. 19 ). Most genic promoters harbouring H3K27me3 in male PGCs are also marked in females and vice versa, with approximately two-thirds of those also marked in ESCs ( Supplementary Fig. 7 ). Interestingly, a relatively large number of promoters (~1,500) are enriched for H3K27me3 exclusively in female PGCs, while a smaller proportion (~270) are enriched exclusively in male PGCs. While most of the genes marked in a sex-specific manner are silenced in both male and female PGCs, we identified a subset of sex-specific H3K27me3-marked genes that show an inverse relationship with expression in PGCs ( Fig. 4c–e and Supplementary Tables 1 and 2 ). In accordance with female E13.5 PGCs preparing to initiate meiosis I and male PGCs undergoing mitotic arrest [22] , [23] , several meiotic genes, including Lfhg and Stra8 (ref. 24 ), show a higher level of expression in female PGCs and, conversely, a higher level of H3K27me3 in male PGCs ( Supplementary Fig. 8 and Supplementary Tables 1 and 2 ). On the other hand, only a small number of male-specific genes, including transforming growth factor-β receptor binding factors Lefty1 and Lefty2 , are marked by H3K27me3 in female PGCs exclusively ( Supplementary Fig. 8 and Supplementary Tables 1 and 2 ), consistent with the recent observation that Nodal signalling is activated specifically in males [25] . Taken together, these results reveal that at this stage in PGC development, the polycomb pathway may be engaged more frequently in the male germ line to regulate germ cell-specific genes. 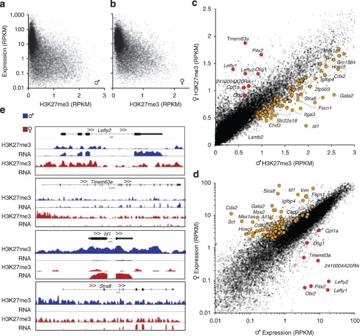Figure 4: Gender-specific H3K27me3 profiles from E13.5 PGCs isolated from single embryos. Relationship between gene promoter enrichment of H3K27me3 (RPKM, RefSeq TSS ±1 kb) and gene expression (exonic RPKM) in male (a) and female (b) E13.5 PGCs. Enrichment of H3K27me3 in genic promoter regions (RPKM, RefSeq TSS ±1 kb) (c) and expression (exonic RPKM) of annotated genes (d) in male versus female PGCs. H3K27me3-marked genes that show an inverse relationship with expression in male (gold) and female (red) PGCs are highlighted. (e) Genome browser screenshots of male versus female H3K27me3 enrichment and gene expression at selected loci, revealing sex-specific H3K27me3-associated gene silencing in E13.5 PGCs. Figure 4: Gender-specific H3K27me3 profiles from E13.5 PGCs isolated from single embryos. Relationship between gene promoter enrichment of H3K27me3 (RPKM, RefSeq TSS ±1 kb) and gene expression (exonic RPKM) in male ( a ) and female ( b ) E13.5 PGCs. Enrichment of H3K27me3 in genic promoter regions (RPKM, RefSeq TSS ±1 kb) ( c ) and expression (exonic RPKM) of annotated genes ( d ) in male versus female PGCs. H3K27me3-marked genes that show an inverse relationship with expression in male (gold) and female (red) PGCs are highlighted. ( e ) Genome browser screenshots of male versus female H3K27me3 enrichment and gene expression at selected loci, revealing sex-specific H3K27me3-associated gene silencing in E13.5 PGCs. Full size image We present a rapid, ULI-NChIP-seq procedure, which can be carried out with as few as 10 3 cells, without sacrificing complexity or resolution [5] , [6] , [7] , [8] , [9] , [10] . Despite the small input size, libraries generated with this method show high resolution and complexity comparable to libraries built with 10 6 cells. Indexing and pooling multiple libraries per sequencing lane not only minimizes sequencing costs but also eliminates the need for pre-amplification of raw ChIP material, which in combination with low PCR cycles at the library construction step reduces the fraction of duplicates and unaligned reads generated. Moreover, the protocol presented here is flexible, allowing freezing, storing and pooling of samples prepared on different days, a valuable feature when working with in vivo samples. ULI-NChIP-seq may also be useful for analysis of non-histone proteins, including transcription factors, that can be immmunoprecipitated in the absence of crosslinking [26] . Using this ULI-NChIP-seq method, we generated H3K27me3 libraries in PGCs isolated from single male and female embryos [19] . While these data sets are correlated with previously published data generated from PGCs pooled from multiple embryos [12] , [13] , ULI-NChIP-seq data sets show improved resolution and a reduced proportion of reads flagged as duplicates, highlighting the benefit of minimizing the number of library amplification cycles and paired-end sequencing. Intersection of our high-resolution NChIP-seq libraries with low-input RNA-seq profiles allowed us to identify a subset of differentially expressed genes that are marked in a sex-specific manner by H3K27me3 in E13.5 PGCs, including both previously identified targets of polycomb group (PcG)-dependent silencing and novel candidates. While it is possible to pool rare samples to generate ChIP-seq libraries, obtaining sufficient cell numbers for previously published ‘low-input’ protocols (>10 4 cells) can be impractical. For example, in our recently published study [19] , only ~3 × 10 3 and ~6 × 10 3 SSEA1+PGCs could be purified by fluorescence-activated cell sorting (FACS) from single male and female wild-type embryos, respectively. In genetically manipulated animals, cell viability can be impacted, decreasing sample yield yet further. Furthermore, embryos with the desired genotype may represent only a small fraction of each litter, so the ULI-NChIP-seq method presented here minimizes the breeding colony size required for genome-wide analyses. As multiple histone marks can be profiled simultaneously with transcription in individual embryos, the variability inherent in studies of cell types that are in the process of transcriptional reprogramming in association with developmental stage is also minimized. ULI-NChIP-seq should also be useful for studies of clinical samples, where cell numbers are frequently limiting. Cell culture and isolation TT2 mouse ESCs [27] were cultured in DMEM supplemented with 15% fetal bovine serum (HyClone), 20 mM HEPES, 0.1 mM non-essential amino acids, 0.1 mM 2-mercaptoethanol, 100 U ml −1 penicillin, 0.05 mM streptomycin, leukemia inhibitory factor and 2 mM L -glutamine on gelatinized plates. Trypsinized cells were either FACS-sorted or aliquoted in nuclear isolation buffer (Sigma, N3408) containing protease inhibitor cocktail (Roche), flash-frozen and stored at −80 °C for a few weeks to a few months. ‘Gold-standard’ NChIP For ‘gold-standard’ NChIP [14] , [16] , 10 6 cells were resuspended in douncing buffer (10 mM Tris-HCl, pH 7.5, 4 mM MgCl 2 , 1 mM CaCl 2 and protease inhibitor cocktail) and homogenized through a syringe. Chromatin was digested in 2 U μl −1 MNase (Worthington Biochemicals) at 37 °C for 5 min, and the reaction was quenched by 0.5 M EDTA. Chromatin was resuspended in hypotonic buffer (0.2 mM EDTA, pH 8.0, 0.1 mM benzamidine, 0.1 mM phenylmethylsulfonyl fluoride, 1.5 mM dithiothreitol and 1 × protease inhibitor cocktail (PIC) and incubated for 1 h on ice. Cellular debris was pelleted and the supernatant was recovered. Chromatin was pre-cleared with 20 μl of 1:1 protein A:protein G Dynabeads (Life Technologies) and immunoprecipitation was carried out with antibody–bead complexes (5 μl Active Motif no. 39161 H3K9me3 antibody and 20 μl 1:1 protein A:protein G Dynabeads) overnight at 4 °C. IPed complexes were washed twice with 400 μl of ChIP wash buffer I (20 mM Tris-HCl, pH 8.0, 0.1% SDS, 1% Triton X-100, 2 mM EDTA and 150 mM NaCl) and twice with 400 μl of ChIP wash buffer II (20 mM Tris-HCl (pH 8.0), 0.1% SDS, 1% Triton X-100, 2 mM EDTA and 500 mM NaCl). Protein–DNA complexes were eluted in 200 μl of elution buffer (100 mM NaHCO 3 and 1% SDS) for 2 h at 68 °C. IPed material was purified by phenol chloroform and 5 ng of raw ChIP material was processed for library construction. ULI-NChIP A detailed, step-by-step procedure is presented in Supplementary Methods . We based our chromatin preparation on a previously published MNase chromatin fragmentation and library construction from single cells [28] . TT2 mouse ESCs were either FACS-sorted directly in nuclear isolation buffer (Sigma; <20,000 cells) or pelleted and re-suspended in nuclear isolation buffer (Sigma). Depending on input size chromatin was fragmented for 5–7.5 min using MNase at 21 or 37 °C, and diluted in NChIP immunoprecipitation buffer (20 mM Tris-HCl pH 8.0, 2 mM EDTA, 15 mM NaCl, 0.1% Triton X-100, 1 × EDTA-free protease inhibitor cocktail and 1 mM phenylmethanesulfonyl fluoride (Sigma)). Chromatin was pre-cleared with 5 or 10 μl of 1:1 protein A:protein G Dynabeads (Life Technologies) and IPed with 0.25 or 1 mg of H3K9me3 (Active Motif no. 39161), H3K27me3 (Diagenode pAb-069–050) or pan-H3 (Sigma, I8140) antibody–bead complexes overnight at 4 °C. IPed complexes were washed twice with 400 μl of ChIP wash buffer I (20 mM Tris-HCl, pH 8.0, 0.1% SDS, 1% Triton X-100, 0.1% deoxycholate, 2 mM EDTA and 150 mM NaCl) and twice with 400 μl of ChIP wash buffer II (20 mM Tris-HCl (pH 8.0), 0.1% SDS, 1% Triton X-100, 0.1% deoxycholate, 2 mM EDTA and 500 mM NaCl). Protein–DNA complexes were eluted in 30 μl of ChIP elution buffer (100 mM NaHCO 3 and 1% SDS) for 2 h at 68 °C. IPed material was purified by phenol chloroform, ethanol-precipitated and raw ChIP material was re-suspended in 10 mM Tris-HCl pH 8.0. As material obtained after ChIP is minimal, DNA concentration was not measured in samples before library construction. For optimal results, raw ChIP material was re-purified with 1.8 × volume of Ampure XP DNA purification beads (Agencourt) before library construction. RNA extraction and double-stranded cDNA preparation Total RNA was extracted from a frozen 10 3 cells aliquots using TRIzol (Invitrogen, AM9738) according to the manufacturer’s manual. Residual genomic DNA was removed by treatment with DNase I (Promega), and ribosomal RNA was depleted using the RiboMinusTranscriptome Isolation kit (Invitrogen) according the manufacturer’s low-input protocol. First strand cDNA synthesis was carried out using Superscript III (Invitrogen 18080-093) with T4 protein 32 and a combination of random 15-mers and oligo dT (NEB), followed by second strand cDNA synthesis using the Klenow polymerase (NEB) in the presence of RNase H. Double-stranded cDNA was fragmented using a BioRuptor (Diagenode) for 15 min (low power mode, 30 s on and 30 s off). Library construction For ‘gold-standard’ H3K9me3 NChIP-seq, 5 ng of raw ChIP material was used for library construction. For ULI-NChIP-seq, 85% of the raw ChIP material was used for library construction. Illumina libraries were constructed using a modified custom paired-end protocol [28] . In brief, samples were end-repaired (1 × T4 DNA ligase buffer, 0.4 mM dNTP mix, 2.25 U T4 DNA polymerase, 0.75 U Klenow DNA polymerase and 7.5 U T4 polynucleotide kinase; 30 min at 21–25 °C), A-tailed (1 × NEB buffer 2, 0.4 mM dNTPs and 3.75 U of Klenow (exo-); 30 min at 37 °C) and ligated (1 × rapid DNA ligation buffer, 1 mM Illumina PE adapters and 1,600 U DNA ligase; 1–8 h at 21–25 °C). Ligated fragments were amplified using indexed primers (Illumina) for 8–10 PCR cycles. DNA was purified with 1.8 × volume Ampure XP DNA purification beads between each step. Sequencing and alignment Amplified indexed libraries were pooled, size selected on a 2% agarose gel and diluted to a final concentration of 10 mM. Cluster generation and paired-end sequencing (100 bp reads) were performed on the Illumina cluster station and Illumina HiSeq 2000 or Illumina HiSeq 2500 sequencing platforms using Illumina Read 1 and Read 2 primers, and a third custom primer (5′- GATCGGAAGAGCGGTTCAGCAGGAATGCCGAGACCG -3′) to sequence the 6-mer unique index. Sequence reads were mapped to mm9 (NCBI 37) using Burrows-Wheeler Aligner (BWA) [29] , and duplicate reads were marked using Picard-tools ( http://picard.sourceforge.net ). Reads passing Illumina’s default chastity filter (total reads) were used to generate library statistics using Samtools Flagstats [30] , where reads with the exact same sequence are identified as ‘duplicates’, non-duplicate reads with a MapQ>5 are identified as distinct uniquely aligned reads and reads with a MapQ<5 are identified as distinct multi-aligned reads. Data sets ChIP-seq and RNA-seq data sets prepared for this manuscript are available at the Gene Expression Omnibus repository under the accession number GSE63523 . H3K27me3 ChIP-seq data sets prepared from 10 3 male and female E13.5 PGCs using ULI-NChIP-seq [19] , and low-input RNA-seq data sets are available under the accession GSE60377 . ENCODE [18] H3K4me3 data sets generated from E14 ESCs (SRR568477 and SRR568478) and H3K27me3 data sets generated from E13.5 PGCs were obtained from accessions GSE38165 (ref. 13 ) and SRA027978 (ref. 12 ). Data analysis For analysis of relative ChIP enrichment at unique loci, duplicate reads (with identical coordinates) and reads with a MapQ<5 (multi-aligned reads) were removed. Multi-aligned reads were included for calculating the relative ChIP enrichment at agglomerated transposable elements. Normalization of relative ChIP enrichment was calculated as reads per kilobase per million mapped reads (RPKM) [31] , [32] . For mined data sets using short, single-end reads, reads were extended to 300 bp before generating RPKM values. Potential library complexity was determined using the extrapolate function of the PreSeq package [15] . For expression analysis, normalization of RNA-seq read enrichment was calculated as RPKM at exonic regions only (RefSeq transcripts). Peak calling Regions enriched for H3K9me3 or H3K27me3 were determined using MACS and MACS2 peak callers on non-duplicate, uniquely aligned reads [33] , [34] . For H3K9me3 peaks, broad domains were identified using MACS2 broadpeaks ( P value=0.05) and combined with narrow domains identified with MACS (10 5 and 10 6 cells input: P value=0.01; 10 3 and 10 4 cells input: P value=0.02). Peaks closer than 2 kb apart were merged and peaks larger than 0.5 kb were included in our analysis. Similarly, for H3K27me3 peaks, broad regions were called using MACS2 broadpeaks ( P value=0.05) and combined with narrower domains identified with MACS (10 4 and 10 5 cells input: P value-0.01; 10 3 cells input: P value=0.02). Peaks closer than 2 kb apart were merged and peaks larger than 0.5 kb were included in our analysis. How to cite this article: Brind’Amour, J. et al . An ultra-low-input native ChIP-seq protocol for genome-wide profiling of rare cell populations. Nat. Commun. 6:6033 doi: 10.1038/ncomms7033 (2015). Accession codes : ChIP-seq and RNA-seq data sets prepared for this manuscript are available at the Gene Expression Omnibus (GEO) repository under the accession number GSE63523 . Referenced data sets:GEO repository: GSE60377 , GSE38165 . Sequence Read Archive (SRA) repository: SRA027978 , SRR568477 and SRR568478 .